Transition-metal-substituted polyoxometalate derivatives as functional anti-amyloid agents for Alzheimer’s disease Inhibitions of amyloid β (Aβ) aggregation and Aβ-haem peroxidase-like activity have received much attention because these two symptoms can be the primary targets of therapeutic strategies for Alzheimer’s disease (AD). Recently, our group found that polyoxometalate (POM) with a Wells–Dawson structure can efficiently inhibit Aβ aggregation. However, the interaction between POMs and Aβ is robust, but still needs to improve Aβ binding affinity. More importantly, it is unclear whether POMs can cross the blood–brain barrier and decrease Aβ-haem peroxidase-like activity. Here we show that our designed series of transition metal-functionalized POM derivatives with a defined histidine-chelated binding site have much better Aβ inhibition and peroxidase-like activity inhibition effects than the parent POM. More intriguingly, we show that these compounds can cross the blood–brain barrier and are metabolized after 48 h. Our work provides insights into the design, synthesis and screening of inorganic metal compounds as multifunctional therapeutic agents against AD. Alzheimer’s disease (AD) is characterized by cerebral extracellular amyloid plaques and intracellular neurofibrillary tangles [1] . Although the molecular mechanisms of AD pathogenesis are not clearly understood owing to its complexity, recent studies have demonstrated that the polymerization of amyloid β-peptides (Aβ) into amyloid fibrils is crucial [1] , [2] , [3] . Therefore, the design, synthesis and screening of Aβ aggregation inhibitors have received much attention for the therapeutic and preventive treatment of AD. Since the discovery of the antitumor activity of cisplatin, a number of inorganic metal compounds have been used as important therapeutic agents and diagnostic imaging probes [4] , [5] , [6] , [7] , [8] , [9] , [10] , [11] , [12] , [13] , [14] , [15] . Worldwide sales of inorganic drugs are rapidly increasing. However, few inorganic agents have been reported that can inhibit Aβ amyloid formation [6] , [7] , [8] , [9] , [10] , [11] . Polyoxometalates (POMs) are early transition metal oxide clusters (especially Mo, W and V) with high oxidation states, and they are used for constructing molecular architectures with potential applications [16] , for example, in catalysis [17] , magnetic materials [18] , chiral recognition [19] or nanocomposites [20] . Furthermore, POMs are promising candidates for drug-carrier approaches on the way to new composite drugs because they have long been known for their multifaceted bioactivity that encompasses antiviral, anticancer, antibacterial and herbicidal properties [21] . Some functionalized POMs have been used as inhibitors of HIV-1 protease [21] or the DNA-binding activity of Sox2 (ref. 22) [22] . Most recently, our group has reported that POMs can be excellent inhibitors to the aggregation of Aβ, and, among them, the phosphotungstate with a Wells–Dawson structure (POM-Dawson) has the strongest inhibition effect [23] . However, the interactions between POMs and Aβ are mainly dependent on favourable electrostatic attraction and POM size effects, which are robust but not specific. For increasing the specificity of POMs binding to Aβ with improved cytotoxicity, it is important and feasible to modify POM-Dawson by introducing a specific Aβ recognition factor. According to previous results, POMs target the cationic cluster from His13 to Lys16 (HHQK) on Aβ [23] . Notably, this cluster contains two adjacent histidines, which can specifically chelate transition metal ions, such as Ni(II) or Co(II) [24] , [25] , [26] , [27] . Therefore, histidine can be a potential chelating site for POMs to improve their specific recognition of Aβ. As a result, POMs with a defined histidine-chelating site may enhance their Aβ inhibition effects. Moreover, it was not safe enough when Aβ peptides were just inhibited, since recently it has been reported that haem binds to Aβ monomers, which may play another major role in AD. The Aβ–haem complex is shown to be a peroxidase, which catalyses the oxidation of serotonin and 3,4-dihydroxyphenylalanine by reactive oxygen species. In the native human Aβ peptides, either His13 or His14 can coordinate to haem and His13 probably binds haem specifically. Mutating the His13 and His14 residues simultaneously can prohibit haem binding, inducing loss of peroxidase-like activity [28] , [29] , [30] . Therefore, a strong affinity between an inhibitor and His13 and His14 will suppress the peroxidase-like activity, which could potentially be useful in the treatment of AD. Moreover, few inorganic agents have been reported that can inhibit the Aβ–haem peroxidase-like activity [28] , [30] . However, it is unclear whether transition metal substitution in POM will reveal the best effects. We therefore introduced a semi-rational design approach for our studies. A semi-rational design is a widely used intermediate approach that involves the identification of important residues in a biological enzyme [31] . Here, we describe a series of transition metal-functionalized POM-Dawson derivatives (POMds) with various well-known histidine-chelating metals (such as Cu, Fe, Ni, Co and Mn) ( Fig. 1 ) by using high-throughput screening to verify the improvement in the binding affinity of the POMds to Aβ. As designed, POMds would have much better capability to inhibit Aβ fibril formation and Aβ-mediated peroxidase-like activity. In this way, POMds may act as inorganic dual-functional anti-Aβ agents for the therapy of AD. 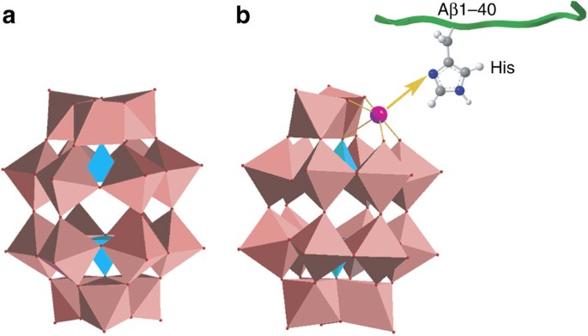Figure 1: Structures of POM and POMds. (a) Wells–Dawson structure; (b) Wells-Dawson POMds with defined histidine-chelating metals (such as Ni, Co, Cu, Fe and Mn). The PO4and WO6polyhedra are shown in blue and light pink, respectively. The histidine-chelating metal is shown as a purple ball. The O, C, N and H atoms are shown as red, grey, dark blue and white balls, respectively. Figure 1: Structures of POM and POMds. ( a ) Wells–Dawson structure; ( b ) Wells-Dawson POMds with defined histidine-chelating metals (such as Ni, Co, Cu, Fe and Mn). The PO 4 and WO 6 polyhedra are shown in blue and light pink, respectively. The histidine-chelating metal is shown as a purple ball. The O, C, N and H atoms are shown as red, grey, dark blue and white balls, respectively. Full size image Characterizations of POM and POMds All POM-Dawson and POMds were synthesized and characterized as previously described ( Supplementary Figs 1,2 and Supplementary Tables 1,2 ) [32] . To identify the capabilities of POM-Dawson and five POMds in inhibiting Aβ aggregation, a high-throughput screening method was used. The screen used a fusion of Aβ42 to enhanced cyan fluorescent protein (Aβ-ECFP). In the absence of inhibition, the rapid misfolding and aggregation of Aβ42 causes the entire fusion protein to misfold, thereby preventing fluorescence. Compounds that inhibit Aβ42 aggregation enable CFP to fold into its native structure and be identified by the resulting fluorescent signal ( Fig. 2 ) [33] . By using this system constructed in our laboratory [23] , we identified POM-Dawson and five POMds capable of inhibiting Aβ aggregation ( Fig. 2 ). All six compounds could increase the fluorescence, indicating that they prevented Aβ aggregation; among the five POMds, only POMds with Ni or Co showed better inhibitory effects than those of unmodified POM-Dawson ( Fig. 3 ). This could be explained as the following. As POM-Dawson targets the HHQK cluster of Aβ [23] , and Ni and Co are well known to possess high binding affinity to histidine [24] , [25] , [26] , [27] , Ni- or Co-metalized POMds would possess better inhibitory effects. On the basis of the screening results, K 8 P 2 NiW 17 O 61 (POMds-Dawson-Ni) and K 8 P 2 CoW 17 O 61 (POMds-Dawson-Co) were used in the following studies. 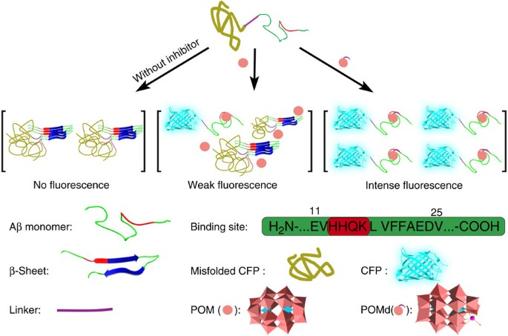Figure 2: Schematic illustration of the high-throughput screening method for identifying effective Aβ-aggregation inhibitors. In the absence of inhibitors, the Aβ42 portion of the fusion aggregates rapidly and causes the entire Aβ42–ECFP fusion to misfold and aggregate (left). Therefore, no fluorescence is observed. However, inhibition of Aβ42 aggregation enables CFP to form its native fluorescent structure (middle, right). Figure 2: Schematic illustration of the high-throughput screening method for identifying effective Aβ-aggregation inhibitors. In the absence of inhibitors, the Aβ42 portion of the fusion aggregates rapidly and causes the entire Aβ42–ECFP fusion to misfold and aggregate (left). Therefore, no fluorescence is observed. However, inhibition of Aβ42 aggregation enables CFP to form its native fluorescent structure (middle, right). 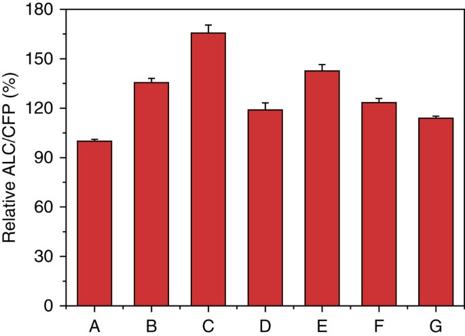Figure 3: ECFP-based screening of Aβ aggregation inhibitors in livingE. colicells. A to G: control (without POMs), Dawson-POM, Dawson-POM-Ni, Dawson-POM-Mn, Dawson-POM-Co, Dawson-POM-Cu, Dawson-POM-Fe. % ALC/CFP means percentage of the fluorescence intensity ofE. colicells expressing ALC divided by the fluorescence ofE. colicells expressing CFP. Data represent the average of three replicate experiments and the error bars indicate the ±s.d. Full size image Figure 3: ECFP-based screening of Aβ aggregation inhibitors in living E. coli cells. A to G: control (without POMs), Dawson-POM, Dawson-POM-Ni, Dawson-POM-Mn, Dawson-POM-Co, Dawson-POM-Cu, Dawson-POM-Fe. % ALC/CFP means percentage of the fluorescence intensity of E. coli cells expressing ALC divided by the fluorescence of E. coli cells expressing CFP. Data represent the average of three replicate experiments and the error bars indicate the ±s.d. Full size image Stability of POM and POMds One issue that needs to be addressed is the stability of the POM and POMds under our experimental conditions [23] . Thus, the stability of POM-Dawson, POMds-Dawson-Ni and POMds-Dawson-Co was studied by using UV/Vis spectroscopy ( Supplementary Fig. 3 ), mass spectrometry (MS) ( Supplementary Fig. 4 ) and 31 P NMR spectroscopy ( Supplementary Fig. 5 ). The results indicated that all of the POM and POMds used remained intact [23] , [32] . Furthermore, the stabiliy of POM and POMds in the presence of Aβ was also determined by using matrix-assisted laser desorption/ionization time-of-flight (MALDI-TOF) MS ( Supplementary Fig. 6 ). The results indicated that all the POM/POMds and Aβ peptides remained intact. Inhibitory effects of POMds on Aβ aggregation To verify the inhibitory effects of POMds metallated with Ni or Co on Aβ aggregation, we used a commonly used in vitro thioflavin T (ThT) fluorescence assay to perform further studies [23] . ThT, an extrinsic fluorescent dye, is able to bind to amyloid aggregates; upon binding, its fluorescence intensity increases. The formation of amyloid fibrils was quantified by measuring the fluorescence intensity of ThT at 480 nm upon excitation at 444 nm, and POM alone did not affect the ThT fluorescence under our experimental conditions. When fresh Aβ1-40 was incubated alone at 37 °C, the ThT fluorescence, as a function of the incubation time, showed a sigmoidal shape. This result was consistent with the nucleation-dependent polymerization model [34] , [35] , [36] , [37] . However, in the presence of POMds-Dawson-Ni or POMds-Dawson-Co the ThT fluorescence was hardly changed, especially for POMds-Dawson-Ni, indicating that the formation of Aβ amyloid fibrils was suppressed ( Fig. 4a ). The inhibitory effect followed the order POMds-Dawson-Ni>POMds-Dawson-Co>POM-Dawson, which was in agreement with the high-throughput screening results. To compare the inhibitory effects, a previously reported pentapeptide-based fibrillogenesis inhibitor, LPFFD [38] , was used as a positive control ( Supplementary Fig. 7 ). The inhibitory effect of LPFFD was lower than those of all POM and POMd inhibitors. Furthermore, after incubation for 7 days, gel electrophoresis indicated that Aβ1–40 in the absence of POMds had aggregated into higher-order oligomers and fibrils ( Fig. 4b , lane 2) [39] , [40] . In contrast, the formation of Aβ aggregates was markedly inhibited by POMds-Dawson-Co or POMds-Dawson-Ni, as shown by a stronger monomer band and a weaker aggregate band in the native gel ( Fig. 4b , lanes 4, 5), indicating that Aβ aggregation was inhibited. 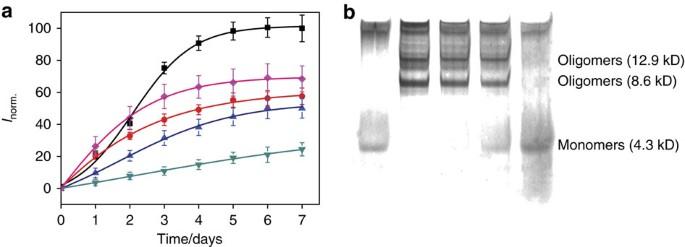Figure 4: Inhibition of Aβ assembly by POMds. (a) Aggregation kinetics of Aβ 1–40 monitored by ThT fluorescence in the absence of POMs/POMds (▪) or the presence of POM-Dawson (▴), POMds-Dawson-Co ([cirf ]) or POMds-Dawson-Ni (▾). The data represented the means of three independent experiments. In contrast, we also tested the inhibition effect when POM-Dawson and Ni2+were just mixed together (□). Error bars indicate ±s.d. (b) Determination of the POMds on the formation of Aβ fibrils by native PAGE. Lane 1: control 1 (Aβ monomer only), lane 2: control 2 (Aβ 1–40 after incubation for 7 days), lane 3: Aβ1–40/ POM-Dawson, lane 4: Aβ1–40/POMds-Dawson-Co, lane 5: Aβ1–40/POMds-Dawson-Ni. Figure 4: Inhibition of Aβ assembly by POMds. ( a ) Aggregation kinetics of Aβ 1–40 monitored by ThT fluorescence in the absence of POMs/POMds (▪) or the presence of POM-Dawson ( ▴ ), POMds-Dawson-Co ([cirf ]) or POMds-Dawson-Ni ( ▾ ). The data represented the means of three independent experiments. In contrast, we also tested the inhibition effect when POM-Dawson and Ni 2+ were just mixed together (□). Error bars indicate ±s.d. ( b ) Determination of the POMds on the formation of Aβ fibrils by native PAGE. Lane 1: control 1 (Aβ monomer only), lane 2: control 2 (Aβ 1–40 after incubation for 7 days), lane 3: Aβ1–40/ POM-Dawson, lane 4: Aβ1–40/POMds-Dawson-Co, lane 5: Aβ1–40/POMds-Dawson-Ni. Full size image We also investigated the effects of POMds-Dawson-Ni and POMds-Dawson-Co on the morphology of Aβ aggregates using atomic force microscopy (AFM) [39] , [40] . Forty micromolar Aβ was incubated in the absence or presence of POMds-Dawson-Ni or POMds-Dawson-Co in buffer (10 mM HEPES, 150 mM NaCl, pH 7.4) at 37 °C for 7 days. Aβ formed long unbranched aggregates ( Supplementary Fig. 8 ). In contrast, in the presence of POMds-Dawson-Ni (20 μM), spherical structures with average heights of 2–3 nm were formed. These results further supported the ThT experiments and indicated that POMds-Dawson-Ni could inhibit the formation of Aβ fibrils. To better compare the inhibitory effects of POM-Dawson, POMds-Dawson-Ni and POMds-Dawson-Co, we evaluated their IC 50 values using a ThT assay ( Supplementary Fig. 9 ) [39] , [40] . Table 1 summarizes their IC 50 values. The results indicated that the IC 50 values of POMds-Dawson-Ni and POMds-Dawson-Co were approximately 4.5-fold and 1.7-fold lower than that of POM-Dawson, respectively ( Table 1 ). In contrast, the peptide LPFFD was also used as a positive control. The IC 50 value of LPFFD (15.60±1.79 μM) (error bars indicate ±s.d., see Supplementary Fig. 9 ) was similar to that of POMds-Dawson-Co and higher than that of POMds-Dawson-Ni. The results suggested that the inhibition efficiency of POMds-Dawson-Ni and POMds-Dawson-Co was significantly increased due to the strong chelation between Ni or Co and the histidine of HHQK. The order of the inhibitory effects followed POMds-Dawson-Ni>POMds-Dawson-Co>POM-Dawson. This order was consistent with our quantitative thermodynamics results. Table 1 Analysis of florescence titration, ITC and IC 50 data. Full size table Recent evidence suggests that amyloid oligomers, which represent intermediates in the fibril formation process, are the main source of cytotoxicity by causing the death of neurons for amyloid pathogenesis, rather than the mature fibrils that accumulate as large aggregates [41] , [42] . To verify the feasibility of the POMds for AD therapeutic applications, we studied their inhibitory effects on Aβ oligomers. The metal-induced oligomer of Aβ was prepared by treatment with Cu 2+ at 37 °C for 24 h and determined by a native polyacrylamide gel electrophoresis (PAGE) assay ( Supplementary Fig. 10 ) [42] . Lane 2 in Supplementary Fig. 10 shows that Aβ treated with Cu 2+ alone had almost no monomer band. In contrast, Aβ oligomer formation was markedly inhibited by coincubating with POMds-Dawson-Co or POMds-Dawson-Ni, as shown by a stronger monomer band and a weaker aggregate band in the native gel ( Supplementary Fig. 10 , lanes 3–5). These findings indicated that Aβ oligomer aggregation was clearly inhibited and POMds-Dawson-Ni showed better effects. To confirm the above electrophoresis results, metal-induced Aβ oligomers were studied by AFM ( Supplementary Fig. 11 ). In the Aβ sample with Cu 2+ , a considerable amount of amorphous aggregates approximately 7 nm in size was detected after 24 h of incubation. While in the presence of POMds-Dawson-Co or POMds-Dawson-Ni, the Aβ oligomer was strongly inhibited, which could be observed as approximately 1.5 nm globules. Aβ monomers were determined as approximately 1.3 nm globules [43] , whereas POMs could hardly be detected by AFM. The binding site and stoichiometry between POMds and Aβ As previously indicated, the binding site on which the initial POM-Dawson located was the cationic cluster HHQK on Aβ [23] . For POMds-Dawson-Co or POMds-Dawson-Ni, the histidine-chelating effect would enhance the POMd binding to HHQK. In order to confirm the existence of the His-chelating effect between the POMds and Aβ monomer, we developed an amino acid-coated Fe 3 O 4 binding assay ( Supplementary Fig. 12A ). For these experiments, a series of Fe 3 O 4 coated with either glycine (Fe 3 O 4 @Gly), valine (Fe 3 O 4 @Val) or histidine (Fe 3 O 4 @His) was synthesized because the content of Gly and Val in Aβ are maximum compared with other amino acids. Each Fe 3 O 4 @amino acid was characterized as previously described ( Supplementary Fig. 13 ) [44] . Then, each amino acid-modified Fe 3 O 4 was adequately incubated with different POM derivatives at several different concentrations for 1 h. The intermixtures were then treated with a magnet to separate the Fe 3 O 4 , and the supernatant was measured at 210 nm, which is the optimal absorption wavelength of POMs [23] . According to the concentration curves of POM and POM derivatives in the supernatant ( Supplementary Fig. 12B ), Fe 3 O 4 @Gly and Fe 3 O 4 @Val hardly bound to the POM derivatives, indicating that the POM derivatives could not be located on these amino acid sites in Aβ. Due to electrostatic attraction effect, Fe 3 O 4 @His could bind to the POM derivatives. However, the affinities of the POMds were obviously stronger than that of POM-Dawson, especially for POMds-Dawson-Ni. Therefore, besides the electrostatic attraction, His-chelating effect also made favourable contribution. The above results suggested that the His-chelating effect did exist between the POMds and Aβ. When the POMds interacted with Aβ, they were prone to being located on the His sites in Aβ, especially on the HHQK cationic cluster because this site contained two adjacent histidines. The stoichiometry for the complexation of POM/POMds with Aβ was first investigated by using Job’s continuous variation method ( Supplementary Fig. 14 ) [45] . The intersection point appeared at 0.5 in the plot, indicating that the binding stoichiometry of the POM/POMds bound to Aβ was 1:1. MALDI-TOF MS was also used to study the POMds binding to Aβ. After incubation of the POMds and Aβ together at 4 °C for 60 min, the unique peak of the POMds–Aβ complex could be easily detected, and the molecular weight was just equal to one POMds plus one Aβ peptide ( Supplementary Fig. 6A ). Under the same conditions, the peak of the POM–Aβ complex was lower than that of the POMds–Aβ compound ( Supplementary Fig. 6B,C ). The results indicated that the POM/POMds bound to Aβ at a 1:1 ratio, and that the POMd binding to Aβ was stronger, which was verified by our next quantitative fluorescence titration experiments. Next, we carried out an enzymatic digestion experiment with trypsin to investigate whether POM derivatives were located at the HHQK cluster on Aβ. Trypsin exclusively cleaves the C-terminal to arginine (R) and lysine (K) residues. We used the shorter fragment Aβ12–28 with the sequence VHHQKLVFFAEDVGSNK, in which the enzyme digestion site and the POM derivatives binding site were at the same sequence. SDS–PAGE electrophoresis was used to determine whether Aβ was digested. The results showed that single Aβ was almost completely degraded after 10 min, whereas in the presence of POM-Dawson, POMds-Dawson-Co or POMds-Dawson-Ni at a 1:2 molar ratio with Aβ, proteolysis was weakened ( Supplementary Fig. 15 ). Specifically, in the presence of POMds-Dawson-Ni, the trypsin-induced degradation of lysozymes was barely affected. These results indicated that POM-Dawson, POMds-Dawson-Co and POMds-Dawson-Ni could interact with the Aβ monomer and protect it from trypsin-induced degradation, and that POMds-Dawson-Ni provided the best protection. Furthermore, the POM derivatives were bound on the cationic cluster HHQK, which might play an important role in the specific binding of POM derivatives with Aβ. The above two results indicated that when interacted with Aβ, POMds would bind to the HHQK cluster because this site was both positively charged and possessed His residues. These results were consistent with previous studies [23] . Molecular dynamic simulations provided further support for their binding. The geometry optimization algorithm was applied for each starting condition; molecular dynamic simulations were then conducted using Autodock Vina until a stable complex was obtained [46] . The best-fit obtained with this method is shown in Fig. 5 . The POM-binding site of Aβ was identified as a cavity-like domain mainly encompassing the amino acids His13, Gln15 and Lys16 of Aβ1−40. This domain of Aβ formed a relatively positively charged surface ( Fig. 5b ), which allowed the interactions with the negatively charged POM. The complex was further stabilized by two hydrogen bonds that involved His13-POM and Arg16-POM ( Fig. 5c ). This result also explained why POM did not bind at His6. There was no existing suitable cavity for recognizing POM around His6, and the amino acids around His6 were all negatively charged (such as Glu3, Asp7 and Ser8), which interfered with the interaction between His6 and POM ( Fig. 5a ). 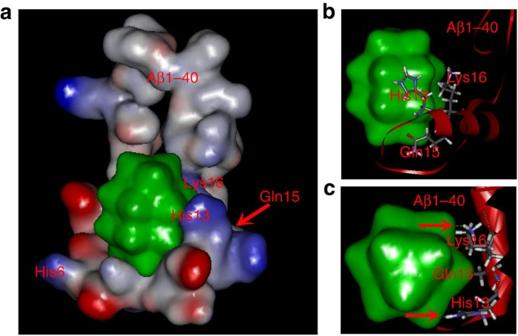Figure 5: Energy-minimized average model of POM-Aβ interactions. This complex is shown in molecular surface models (a) and a tube representation (b,c) with POM in green. A remarkable feature of the model is that the POM-binding site of Aβ is identified as a positive electricity cavity-like domain mainly encompassed by His13, Gln15, Lys16 of Aβ1–40. This is particularly visible in panel B. The complex is further stabilized by two hydrogen bonds, involving His13-POM and Arg16-POM. This is illustrated incby arrows. Figure 5: Energy-minimized average model of POM-Aβ interactions. This complex is shown in molecular surface models ( a ) and a tube representation ( b , c ) with POM in green. A remarkable feature of the model is that the POM-binding site of Aβ is identified as a positive electricity cavity-like domain mainly encompassed by His13, Gln15, Lys16 of Aβ1–40. This is particularly visible in panel B. The complex is further stabilized by two hydrogen bonds, involving His13-POM and Arg16-POM. This is illustrated in c by arrows. Full size image Fluorescence titrations [23] , [39] , [40] were used to estimate the binding constants of POM-Dawson, POMds-Dawson-Co and POMds-Dawson-Ni, which reflected the specificity between inhibitors and Aβ. With increasing POMds-Dawson-Ni or POMds-Dawson-Co, the fluorescence intensity of Aβ was quenched much stronger than that of POM-Dawson ( Supplementary Fig. 16 ). The apparent binding constants, K a , yielded by nonlinear least-squares fit [39] , [40] showed that the K a values of POMds-Dawson-Ni and POMds-Dawson-Co were approximately 6.44 and 3.52 times higher than that of POM-Dawson, respectively ( Table 1 ). Furthermore, the binding free energy change was also estimated ( Table 1 ). The binding free energy difference was approximately 4.6 kJmol −1 between POMds-Dawson-Ni and POM-Dawson. Together, these results indicated that Ni or Co in POMds could enhance their binding affinity and recognition to Aβ with a defined binding site and improve the inhibition efficiency. The stoichiometry and binding constant between POMds and Aβ were confirmed by isothermal titration calorimetry (ITC; Fig. 6 ) [47] , [48] . The binding was exothermic and best fit to a 1:1 binding model. Furthermore, the ITC data demonstrated that the binding constants of the POM-Dawson–Aβ, POMds-Dawson-Co–Aβ and POMds-Dawson-Ni–Aβ complexes were 2.01 × 10 5 , 9.07 × 10 5 and 1.68 × 10 6 , respectively. The binding free energy difference was approximately 5.26 kJmol −1 between POMds-Dawson-Ni and POM-Dawson, which indicated a higher affinity between POMds and Aβ. These results were consistent with the fluorescence titration data ( Table 1 ). 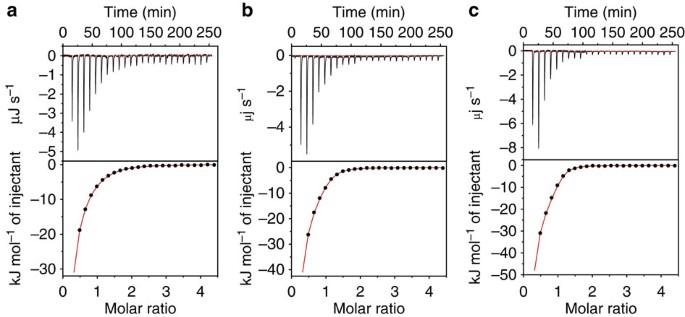Figure 6: Representative ITC data for the interactions between POM/POMds and Aβ. ITC titration curves of POM-Dawson (0.448 mM,a), POM-Dawson-Co (0.448 mM,b) and POM-Dawson-Ni (0.448 mM,c) with Aβ (0.02 mM) at 25 °C. Best-fit ITC values are listed inTable 1. Figure 6: Representative ITC data for the interactions between POM/POMds and Aβ. ITC titration curves of POM-Dawson (0.448 mM, a ), POM-Dawson-Co (0.448 mM, b ) and POM-Dawson-Ni (0.448 mM, c ) with Aβ (0.02 mM) at 25 °C. Best-fit ITC values are listed in Table 1 . Full size image The binding site between Aβ and POMds has been demonstrated to be the cationic cluster HHQK, not His or other single amino acids. The enhanced specific recognition between POMds and Aβ could be attributed to two aspects. First, it was certainly attributed to the increased electrostatic attraction [49] . Because POM-Dawson had six negative charges and the POMds had eight, the additional negative charges could increase the electrostatic attraction towards the cationic cluster HHQK. Second, it could be the histidine-chelating effect, which improved the ability of the POMds to recognize the HHQK cluster. It was clearly observed that, although POMds-Dawson-Co and POMds-Dawson-Ni had the same charges, the electrophoretic mobility of Aβ incubated with POMds-Dawson-Ni was slower. Also, the value of the apparent binding constant K a of POMds-Dawson-Ni was larger than that of POMds-Dawson-Co. These results demonstrated that the His-chelating effect between POMds and HHQK existed and that POMds-Dawson-Ni had the strongest interaction. According to all of the effects mentioned above, POMds-Dawson-Ni showed the best specificity towards Aβ. There are two possible mechanisms by which POMds could inhibit Aβ aggregation more efficiently. The intense binding caused by electrostatic and histidine-chelating effects between POMds and the Aβ monomer would substantially lower the concentration of the free monomer and shift the equilibrium away from aggregation. In addition, it is possible that strong interactions between the POMds and Aβ oligomers could result in unfavourable conditions for nucleation and fibril growth through blocking direct contact between Aβ monomers. This situation would lead to the depletion of sub- and near-critical oligomers and to the partial blockage of the kinetic pathway until the surface is saturated and new nuclei can be grown [39] , [40] , [50] . Inhibition of Aβ-mediated peroxidase-like activity and cytotoxicity Furthermore, it has been recently reported that haem binds to Aβ monomers, which may play another major role in AD ( Fig. 7a ) [28] , [29] , [30] . In native human Aβ peptides, simultaneously mutating the His13 and His14 residues can prohibit haem binding and result in the loss of peroxidase-like activity. According to the above results, we took advantage of the electronegative and His-chelated POMds to show that the POMds-Dawson-Ni and POMds-Dawson-Co strongly targeted the HHQK cluster on Aβ, which blocked His13 and His14 simultaneously. Therefore, POMds could be outstanding inhibitors of the above peroxidase-like activity, and this hypothesis was confirmed. As described previously, haem-Aβ complexes showed remarkably enhanced peroxidase-like activity relative to free haem [28] , [29] , [30] . When POM-Dawson was added to the system, the enhanced peroxidase-like activity still existed. However, when POMds-Dawson-Ni or POMds-Dawson-Co was added instead of POMds-Dawson at the same concentration, the enhanced peroxidase-like activity nearly disappeared ( Fig. 7b , Supplementary Fig. 17 ). The results suggested that POMds-Dawson-Ni and POMds-Dawson-Co acted as more effective inhibitors in depressing the Aβ-mediated peroxidase-like activity and they could be dual-functional agents for the treatment of AD. 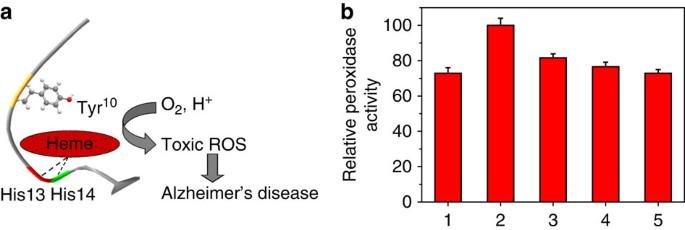Figure 7: Inhibition of Aβ-mediated peroxidase-like activity by POMds. (a) Schematic representation of Aβ-induced peroxidase-like activity generation. The haem-Aβ complexes, in which the haem is coordinated by His13 and His14, have been demonstrated to function as peroxidases. (b) Effect of POMds on the inhibition of Aβ-induced peroxidase-like activity, monitoring the increase of the 420 nm absorbance intensity after 200 s, for different haem-Aβ–POMds complexes: free haem (1); haem+Aβ (2); haem+Aβ+POM-Dawson (3); haem+Aβ+POMds-Dawson-Co (4); haem+Aβ+POMds-Dawson-Ni (5). The experiment was repeated three times. Error bars indicate ±s.d. Figure 7: Inhibition of Aβ-mediated peroxidase-like activity by POMds. ( a ) Schematic representation of Aβ-induced peroxidase-like activity generation. The haem-Aβ complexes, in which the haem is coordinated by His13 and His14, have been demonstrated to function as peroxidases. ( b ) Effect of POMds on the inhibition of Aβ-induced peroxidase-like activity, monitoring the increase of the 420 nm absorbance intensity after 200 s, for different haem-Aβ–POMds complexes: free haem (1); haem+Aβ (2); haem+Aβ+POM-Dawson (3); haem+Aβ+POMds-Dawson-Co (4); haem+Aβ+POMds-Dawson-Ni (5). The experiment was repeated three times. Error bars indicate ±s.d. Full size image Next, we further studied whether POMds-Dawson-Ni and POMds-Dawson-Co could inhibit Aβ-mediated cellular toxicity. To address this question, we used PC12 cells to probe cellular metabolism by using a 3-(4,5-dimethylthiazol-2-yl)-2,5-diphenyltetrazolium bromide (MTT) assay [39] , [40] . Aβ was incubated in the presence or absence of POM-Dawson, POMds-Dawson-Ni or POMds-Dawson-Co for 7 days, and then the cells were exposed to the Aβ/POM mixtures. The data were normalized by using the results for cells not treated with Aβ fibrils as a positive control [39] , [40] . In the presence of POM-Dawson or POMds, the survival of the cells significantly increased ( Fig. 8a ), indicating that POM-Dawson or POMds inhibited Aβ aggregation and decreased Aβ-induced cytotoxicity. POMds had a stronger effect than that of POM-Dawson. POMds-Dawson-Ni showed even better efficiency than POMds-Dawson-Co. At the same time, POM/POMds themselves were nontoxic at the same concentrations ( Fig. 8b ). Thus, POMds-Dawson-Ni and POMds-Dawson-Co could not only inhibit Aβ aggregation during in vitro studies, as evidenced by ThT fluorescence assay, but also decreased Aβ-induced cytotoxicity, which was consistent with our fluorescent live cell screening results. 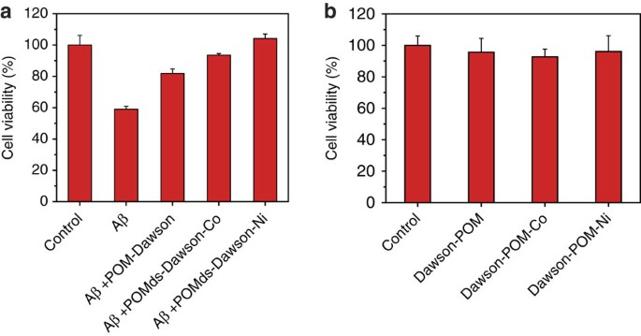Figure 8: Effect of POMds on cell toxicity of Aβ. Samples were prepared in the presence (a) or absence (b) of POM/POMds. The cytotoxic effect on PC12 cells was determined by using MTT assay from three separate measurements. Each experiment had been repeated three times. Error bars indicate ±s.d. Figure 8: Effect of POMds on cell toxicity of Aβ. Samples were prepared in the presence ( a ) or absence ( b ) of POM/POMds. The cytotoxic effect on PC12 cells was determined by using MTT assay from three separate measurements. Each experiment had been repeated three times. Error bars indicate ±s.d. Full size image Blood–brain barrier penetration Due to the excellent profiles against Aβ fibril formation and Aβ-mediated peroxidase-like activity in vitro , POMds may be suitable for generating a bioavailable drug in the treatment of AD. A major impediment to the development of effective anti-Aβ compounds for AD therapy is that essentially 100% of large-molecule drugs and >98% of small-molecule drugs fail to cross the blood–brain barrier (BBB) [51] . To ensure that the POMds could cross the BBB, we treated wild-type mice with POMds-Dawson-Ni, which had the best effect. Each mouse was intravenously administered 25 mg of POMds-Dawson-Ni per kilogram of body weight. Blood and brain tissue were collected at 5, 10, 30 and 60 min post dosing; plasma was then separated from the blood and the brain tissue was homogenized. As a surrogate measure of drug levels, plasma and brain homogenates were analysed for levels of tungsten by inductively coupled plasma mass spectrometry (ICP-MS). As predicted, the levels of W in the plasma rapidly increased to the peak level in the animals treated with POMds-Dawson-Ni after 5 min (approximately 8.91 mg kg −1 ). Notably, the highest level of W in the brain did not appear at the same time as in the plasma, but rather, at 10 min after dosing (approximately 0.0231, mg kg −1 ) ( Supplementary Fig. 18 ). Thereafter, the concentrations of W markedly decreased in both the plasma and brain. After 60 min, only 1.0 and 9.6% of W remained in the plasma and brain, respectively, compared with each peak value. After 48 h, the concentrations of W in both the plasma and brain returned to the initial levels. We used mice treated with only physiological saline as controls; the concentrations of W and Ni in the brains were too low to measure. The in vivo stability of POMds was also evaluated. We treated wild-type Wistar rats with POMds-Dawson-Ni. Each rat was intravenously administered 25 mg of POMds-Dawson-Ni per kilogram of body weight. Brain tissues were collected at 60 min post dosing and homogenized. The brain homogenates were analysed by high-performance liquid chromatography (HPLC). As shown in Supplementary Fig. 19A , the samples had POMds-Dawson-Ni peaks at the same retention time as POMds-Dawson-Ni alone. We also used ICP-MS to study the in vivo stability. The measured Ni/W weight ratio was 1:52.11, and the calculated value was 1:53.25. Both results indicated that POMds-Dawson-Ni was not only permeable but also stable in vivo . Since AD is characterized by cerebral extracellular amyloid plaques, the distribution of POMds in brain tissues should be determined. We treated wild-type Wistar rats with POMds-Dawson-Ni, and each rat was intravenously administered 25 mg of POMds-Dawson-Ni per kilogram of body weight. The cerebrospinal fluids were collected at 60 min after dosing and then centrifuged. The supernatants were also analysed by HPLC. As predicted, the samples had the POMds-Dawson-Ni peaks at the same retention times as those of POMds-Dawson-Ni alone ( Supplementary Fig. 19B ). These findings indicated that POMds-Dawson-Ni could distribute extracellularly in the brain, where Aβ aggregates predominately exist. The HPLC results further confirmed that POM-Dawson-Ni could cross the BBB and remain intact in vivo . In summary, by using a high-throughput screening method based on the fluorescence of an Aβ-ECFP fusion expression system, a ThT fluorescence assay, PC12 cell toxicity and quantitative thermodynamics studies, our designed and synthesized transition metal-functionalized POMds show an improved Aβ inhibitory effect compared with the Wells-Dawson-type POM. A Ni-metallated POM derivative can achieve a sixfold improvement. Transition metal-functionalized POMds with defined histidine-chelated binding sites can not only specifically target the HHQK cluster of Aβ with improved cytotoxicity but also show stronger inhibitory effects through enhanced Aβ binding affinity, as evidenced by the quantitative thermodynamic studies. Moreover, the POMds-Dawson-Ni and POMds-Dawson-Co exhibit better effects for depressing the Aβ-mediated peroxidase-like activity, indicating that our designed and synthesized POMds can be dual-functional therapeutic agents against AD. Furthermore, the POMds can cross the BBB and be metabolized after 48 h. In this sense, our work advances our understanding of the design and synthesis of inorganic metal compounds as multifunctional therapeutic agents against AD. Sample preparation Aβ1-40 was purchased from American Peptide (Sunnyvale, California, USA. lot no. U10012). Peptides were prepared as previously described [23] . Briefly, the powdered Aβ peptide was first dissolved in 1,1,1,3,3,3-hexafluoro-2-propanol at a concentration of 1 mg ml −1 . The solution was shaken at 4 °C for 2 h in a sealed vial for further dissolution and then stored at −20 °C as a stock solution. Before use, the solvent 1,1,1,3,3,3-hexafluoro-2-propanol was removed by evaporation under a gentle stream of nitrogen, and the peptide was dissolved in 10 mM of HEPES buffer (pH 7.4, containing 150 mM of NaCl). High-throughout screening of Aβ inhibitors Briefly, the Escherichia coli strain BL21(DE3) was transformed by the vector ALC (Aβ-linker-ECFP) or the control vector CFP (linker-ECFP) and cultured at 37 °C in lysogeny broth (LB, pH 7.4) containing ampicillin (50 μg ml −1 ). Different POMs or POMds were added to the culture medium 30 min prior to protein expression induced by isopropyl-β-D-1-thiogalactopyranoside (1 mM). After expression of the recombinant proteins for 3 h, all samples were diluted to an optical density of 0.1 at 600 nm. The fluorescence of each sample was measured at 512 nm (excitation 433 nm) with a JASCO FP6500 spectrofluorometer. Compounds were tested in triplicate at a final concentration of 100 μM (ref. 52 ). ThT fluorescence spectroscopy The kinetics of Aβ aggregation was monitored using the dye ThT, the fluorescence of which is dependent on the formation of amyloid fibrils. Fluorescence measurements were carried out with a JASCO FP6500 spectrofluorometer. The fluorescence signal (excitation at 444 nm) was recorded between 460 and 650 nm; 10 nm slits were used for both emission and excitation measurements. The peptide concentration was 1 μM, and the ThT concentration was 10 μM. At different times, aliquots of the Aβ solution were taken for fluorescence measurements. AFM study For the AFM measurements, samples were diluted with deionized H 2 O to yield a final concentration of 1 μM. Next, the sample (20 μl) was applied to freshly cleaved muscovite mica and allowed to dry. Data were acquired in the tapping mode on a Nanoscope V multimode atomic force microscope (Veeco Instruments, USA). The resonance frequency was 358.305 Hz, and the scanning frequency was 0.996 Hz. Homoeothermic equipment was used to maintain the temperature during the scan. Native gel electrophoresis Samples (10 μl) were analysed by 12% native PAGE. Gels were run in a Tris/glycine system and developed by the silver-stain method. Fluorescence titration The binding constants of POMds with Aβ were determined by fluorescence titration at 25 °C. The excitation wavelength was 278 nm, and the emission intensity at 306 nm was monitored as a function of continuous increasing concentrations of POMds. The Aβ40 peptide concentration was fixed at 3 μM, whereas the POMds concentration was varied between 0–5.5 μM. The 1:1 binding stoichiometric equation was used to calculate the binding constants [39] , [40] . Amino acid-coated Fe 3 O 4 binding assay To an aqueous solution of a mixture of Fe(III) and Fe(II) salts, an amino acid solution in the molar ratio 2Fe(III):1Fe(II):4 amino acids was added and maintained at a constant temperature of 40 °C for 15 min under vigorous stirring. Next, a solution of ammonium hydroxide was added until the pH was increased to approximately 11, at which point a black suspension formed. This suspension was then refluxed at 80 °C for 6 h under vigorous stirring. The amino acid-coated Fe 3 O 4 were separated from the aqueous solution by magnetic decantation, washed with distilled water several times and then dried in an oven overnight. Each amino acid-modified Fe 3 O 4 was adequately incubated with different POM derivatives at several different concentrations for one hour. The intermixtures were then treated with a magnet to separate Fe 3 O 4 , and the supernatant was measured at 210 nm (ref. 44 ). Trypsin digestion Aβ (20 μM) was preincubated in 10 mM Tris buffer (pH 7.4) in the absence or presence of POM (in 2:1 Aβ/POM ratios) for 30 min at 37 °C; it was then subjected to proteolysis by trypsin (0.1 mg ml −1 ) under the same conditions for 10 min. At the end of the reaction, all samples were supplemented with native PAGE reducing sample buffer, carefully heated at 100 °C for 5 min and subjected to native PAGE (20%). The gels were then silver-stained. Isothermal Titration Calorimetry ITC assays were performed on a NANO ITC System (TA Instruments Inc., New Castle, Delaware, USA). Titrations were performed in buffer (10 mM HEPES buffer, 150 mM NaCl, pH=7.4). Injections of 10 μl of 0.45 mM POM or POMds were added from a computer-controlled microsyringe at an interval of 600 s into an Aβ (20 μM) solution, with stirring at 400 r.p.m. at 25 °C. The experimental data were analysed with NanoAnalyze software (TA Instruments Inc.) and were fitted to an independent model concurrently with a blank constant model to adjust for the heat of dilution. All measurements were obtained from 25 injections of 0.45 mM POM or POMds into 1400 μl of Aβ in 10 mM HEPES, 150 mM NaCl, pH=7.4 buffer at 25 °C. Each heat-burst curve was the result of a 10 μl injection of POM or POMds into the Aβ solution. 31 P NMR and MALDI-TOF MS 31 P NMR spectroscopy measurements were carried out on a Bruker Avance 600 MHz NMR spectrometer at 10 °C. POM samples were dissolved in D 2 O. Experimental conditions were according to Lyou et al . [32] Samples were deposited on the MALDI target using a dried droplet method [24] . MALDI-TOF MS experiments were performed in positive ion mode on an Autoflex III TOF/TOF analyser (Bruker Daltonics Inc., Germany) with the Nd-YAG laser operated at 355 nm with 0 ns duration pulses, a repletion rate of 200 Hz and an acceleration voltage of 19 kV. MS spectra were acquired as an average of 100 laser shots for two times. The laser intensity presented here was defined as 45% of the total laser intensity according to the practical instrument condition. Inhibition of Aβ-mediated peroxidase-like activity and cytotoxicity assays The inhibition assay was performed as previously described [28] , [29] , [30] . Cytotoxicity was measured as follows. PC12 cells (rat pheochromocytoma, American Type Culture Collection) were cultured in Iscove-modified Dulbecco’s medium (Gibco BRL) supplemented with 5% foetal bovine serum and 10% horse serum in a humidified 5% CO 2 environment at 37 °C. Cells were plated at a density of 10,000 cells per well on 96-well plates in fresh medium (90 ml). After 24 h, Aβ1-40 peptides (5 μM) that had been aged with or without POMs were added, and the cells were further incubated for 48 h at 37 °C. Cytotoxicity was measured using a modified MTT assay kit (Promega). The absorbance values of formazan were determined at 490 nm with an automatic plate reader. Blood−brain barrier penetration assay POMds-Dawson-Ni in saline was intravenously administered to wild-type mice through a tail vain injection at 25 mg·kg −1 body weight. Brain tissues were collected at 5, 10, 30 and 60 min after dosing; the plasma was then separated from the blood, and the brain tissue was homogenized. As a surrogate measure of drug levels, the plasma and brain homogenates were analysed for levels of tungsten by ICP-MS [52] . How to cite this article : Gao, N. et al. Transition-metal-substituted polyoxometalate derivatives as functional anti-amyloid agents for Alzheimer’s disease. Nat. Commun. 5:3422 doi: 10.1038/ncomms4422 (2014).